α-Mannosidase 2C1 attenuates PTEN function in prostate cancer cells PTEN dephosphorylates the 3-position phosphate of phosphatidylinositol 3,4,5 triphosphate (PIP 3 ), thereby inhibiting AKT activation. Although attenuation of PTEN function has a major role in tumourigenesis, the underlying mechanisms remain unclear. Here we show that α-mannosidase 2C1 (MAN2C1) inhibits PTEN function in prostate cancer (PC) cells and is associated with a reduction in PTEN function in primary PC. MAN2C1 activates AKT and promotes the formation of PTEN-positive DU145 cell-derived xenograft tumours by imparing endogenous PTEN function. In 659 PC patients who were examined, ∼ 60% of tumours were PTEN positive with elevated AKT activation. Of these, 80% display MAN2C1 overexpression that co-localizes with PTEN. Increases in MAN2C1 were detected only in PTEN-positive prostatic intraepithelial neoplasia and carcinomas, and showed a significant association with PC recurrence only in patients with PTEN-positive PCs. Mechanistically, MAN2C1 binds PTEN thereby inhibiting its PIP 3 phosphatase activity. These findings show that MAN2C1 function as a PTEN-negative regulator in PC cells. PTEN is a phosphatase that functions on both protein and lipid substrates [1] . Accumulating evidence reveals that the lipid phosphatase activity of PTEN, which dephosphorylates the 3-position phosphate from the inositol ring of phosphatidylinositol 3,4,5 triphosphate (PIP 3 ) [2] , [3] , can suppress tumour growth and development. As a result, PTEN directly antagonizes a critical oncogenic event mediated by the phosphatidylinositol-3 kinase (PI3K) [4] , [5] . Typical mechanisms responsible for PTEN inactivation in cancers include genetic and epigenetic events. PTEN +/− mice as well as tissue-specific PTEN knockout mice exhibit a variety of tumours, including lymphoma, liver cancer and lung cancer [6] , [7] . Consistent with these observations, the PTEN gene is frequently mutated in human cancers [8] , [9] , [10] , including over 50% of glioblastomas and melanomas, 30–50% of endometrial carcinomas and 10% of breast cancers [4] , [11] , [12] . A missense mutation PTEN/G129E, leading to loss of the PIP 3 phosphatase activity of the PTEN [4] , [13] , is causative for Cowden disease [14] , a multiple hamartoma syndrome with predisposition to multisystemic malignant tumours [15] . Hypermethylation of the PTEN promoter in sporadic colorectal cancers and reduction of PTEN protein without mutations in the PTEN gene in prostate cancer (PC) also contribute to tumourigenesis [16] , [17] . Loss of PTEN has a critical role in PC progression [13] , [18] . PTEN +/− mice develop prostatic epithelial dysplasia and hyperplasia [19] , [20] , [21] , [22] , [23] . Prostate-specific deletion of PTEN in mice elicits PC that mimics the human condition [24] . This is attributable to the activation of the PI3K/AKT pathway, as loss of AKT1 markedly inhibits the tumourigenesis of prostate and endometrial cancers in PTEN +/− mice [22] . Loss of the PTEN protein has been reported in PC cell lines, in xenografted PCs and more frequently in metastatic PCs [4] , [8] , [18] , [25] . Furthermore, inactivation of PTEN and activation of the PI3K/AKT pathway results in androgen independency in prostate carcinogenesis [26] and inhibition of AKT activity by Psoralidin can overcome chemoresistance in androgen-independent PCs [27] . Potential mechanisms resulting in loss of PTEN function in PC include mutations in the PTEN gene and reduction of the PTEN protein in ∼ 50% of PCs [17] . However, a large proportion of primary PCs express PTEN at normal levels, suggesting that PTEN can be inactivated during prostate tumourigenesis by mechanisms that are neither genetic nor epigenetic. In support of this concept, PTEN function is impaired when expressed at physiological levels in renal cell carcinoma and T-cell acute lymphobastic leukaemia [28] , [29] . These findings strongly suggest that PTEN-mediated tumour suppression can be regulated by additional cellular factors. Consistent with this notion, recent publications show that PTEN is inhibited by binding to Dlg-1 in Schwan cells [30] , and by interacting with P-REX2a and shank-interacting protein-like 1 (SIPL1) in breast and cervical cancers, respectively [31] , [32] . We report here that α-mannosidase 2C1 (MAN2C1) is a novel PTEN-negative regulator (PTEN-NR) in PC cells. MAN2C1 belongs to the α-mannosidase family [33] . Consistent with the family being involved in glycoprotein maturation in the endoplasmic reticulum (ER) and Golgi [34] , MAN2C1 displays mannose-trimming activity [33] . Although MAN2C1 has been reported to be associated with tumourigenic activity in B cells [35] and nasopharyngeal carcinoma [36] , the underlying mechanisms remain unclear. We demonstrate here that MAN2C1 binds to PTEN both in PC cells and in primary PCs, thereby attenuating the PIP 3 phosphatase activity of PTEN and promoting prostate tumourigenesis. Identification of α-MAN2C1 as a PTEN-NR We have recently established a screening approach to select for negative regulators (NRs) of PTEN [32] . Briefly, ectopic PTEN potently inhibited the proliferation of PTEN-deficient LNCaP PC cells, an observation consistent with those reported in glioma, melanoma and breast cancer [2] , [10] , [37] , [38] , and this inhibition was prevented by specific cDNAs derived from a human prostate cDNA library [32] . One of four PTEN-NR cDNAs encoded the last carboxy (C)-terminal 236 residues of MAN2C1 (C-MAN236; Supplementary Fig. S1a ). Although one candidate elicited moderate PTEN inhibitory activity [32] , both SIPL1 [32] and MAN2C1 described in this study potently inhibited PTEN function. To confirm that MAN2C1 attenuates PTEN function, we demonstrated that MAN2C1 enhanced LNCaP cell survival in the presence of ectopic PTEN overexpression in comparison with empty vector (EV; Fig. 1a ). To determine the effect of endogenous MAN2C1 on PTEN function, we first raised an anti-MAN2C1 antibody, which specifically recognizes MAN2C1 ( Supplementary Fig. S1b–d ). By immunoblot analysis using this antibody, we demonstrated knockdown of MAN2C1 using a specific short interfering RNA (siRNA) in PTEN-positive DU145 PC cells ( Fig. 1b ). Knockdown of MAN2C1 decreased cell survival to 30% of control (Ctrl) siRNA-treated cells, which was increased to 75% when PTEN was also knocked down ( Fig. 1c ), demonstrating that knockdown of MAN2C1 significantly inhibited DU145 cell survival/proliferation by enhancement of endogenous PTEN function. This is consistent with endogenous PTEN being functional as knockdown of PTEN increased AKT activation ( Fig. 1b , see AKT-P in PTEN siRNA versus AKT-P in Ctrl siRNA-treated cells). Similar effects were also obtained following MAN2C1/PTEN knockdown using different siRNA fragments that were delivered into DU145 cells through either oligonucleotide or retrovirus methodologies ( Supplementary Table S1 ). In accordance with PTEN antagonism of PI3K-mediated AKT activation, ectopic MAN2C1 enhanced AKT activation in DU145 cells, which was inhibited by the PI3K inhibitor Wortmannin ( Fig. 1d ), but was unable to increase AKT activation in PTEN-negative LNCaP and U87 cells ( Fig. 1e ). These observations suggest that MAN2C1 promotes AKT activation by inhibition of endogenous PTEN function. In further support of this concept, we demonstrated that MAN2C1 siRNA reduced AKT activation in PTEN-positive DU145 ( Fig. 1b ), as well as in MCF7 breast cancer cells ( Supplementary Fig. S2a ), but not in DU145 or MCF7 cells in which endogenous PTEN was concomitantly knocked down ( Fig. 1b , Supplementary Fig. S2a ). Taken together, the above observations demonstrate that MAN2C1 negatively regulates PTEN function. 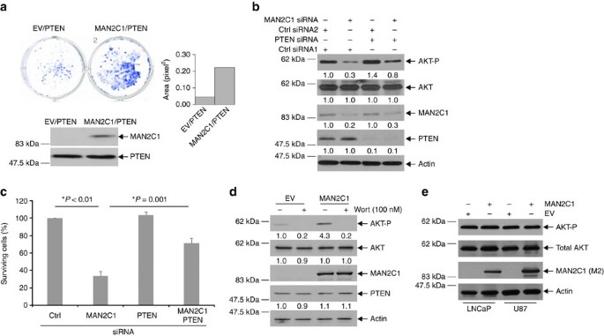Figure 1: MAN2C1 negatively regulates PTEN function. (a) LNCaP cells were infected with EV (empty vector)/PTEN or MAN2C1/PTEN and selected with puromycin for PTEN-retrovirus infection. Surviving cells were stained with crystal violet (top left panels) and quantified (top right panel). Ectopic proteins were demonstrated by western blotting (bottom panel). (b) DU145 cells were infected with a retroviral-based PTEN siRNA or control siRNA (Ctrl siRNA1), followed by transfection with 100 nM MAN2C1 siRNA or its Ctrl siRNA2 for 3 days. The expression of AKT-P (Ser473 phosphorylated AKT), AKT (total AKT), MAN2C1, PTEN and actin were determined by western blot. The levels of individual proteins were quantified against actin and presented under individual panels as fold changes in comparison to Ctrl siRNA-treated cells. (c) Five days after transfection with MAN2C1 siRNA, cell numbers were counted and expressed as percentages of Ctrl siRNA-treated cells. Experiments were repeated three times. Means±standard derivations are shown. *Statistical significance (two-tailed Student'st-test) in the indicated comparisons (Ctrl siRNA versus MAN2C1 siRNA,P<0.001; MAN2C1 siRNA versus MAN2C1 siRNA/PTEN siRNA,P=0.001). (d) DU145 cells were infected with EV or MAN2C1 retrovirus and selected with hygromycin for 48 h to ensure 100% infection. Cells were then treated with DMSO (−) or wortmannin (Wort) for 1 h before western blotting. Experiments were repeated three times and a representative blot is shown. Levels of individual proteins were quantified against actin and presented under individual panels as fold changes in comparison to mock-treated EV cells. (e) LNCaP and U87 cells were infected with EV or MAN2C1 retrovirus, followed by selection with hygromycin for 3 days to achieve 100% transfection and then examined for AKT activation (AKT-P), AKT, ectopic MAN2C1 (using M2 anti-FLAG antibody) or actin by western blotting. Figure 1: MAN2C1 negatively regulates PTEN function. ( a ) LNCaP cells were infected with EV (empty vector)/PTEN or MAN2C1/PTEN and selected with puromycin for PTEN-retrovirus infection. Surviving cells were stained with crystal violet (top left panels) and quantified (top right panel). Ectopic proteins were demonstrated by western blotting (bottom panel). ( b ) DU145 cells were infected with a retroviral-based PTEN siRNA or control siRNA (Ctrl siRNA1), followed by transfection with 100 nM MAN2C1 siRNA or its Ctrl siRNA2 for 3 days. The expression of AKT-P (Ser473 phosphorylated AKT), AKT (total AKT), MAN2C1, PTEN and actin were determined by western blot. The levels of individual proteins were quantified against actin and presented under individual panels as fold changes in comparison to Ctrl siRNA-treated cells. ( c ) Five days after transfection with MAN2C1 siRNA, cell numbers were counted and expressed as percentages of Ctrl siRNA-treated cells. Experiments were repeated three times. Means±standard derivations are shown. *Statistical significance (two-tailed Student's t -test) in the indicated comparisons (Ctrl siRNA versus MAN2C1 siRNA, P <0.001; MAN2C1 siRNA versus MAN2C1 siRNA/PTEN siRNA, P =0.001). ( d ) DU145 cells were infected with EV or MAN2C1 retrovirus and selected with hygromycin for 48 h to ensure 100% infection. Cells were then treated with DMSO (−) or wortmannin (Wort) for 1 h before western blotting. Experiments were repeated three times and a representative blot is shown. Levels of individual proteins were quantified against actin and presented under individual panels as fold changes in comparison to mock-treated EV cells. ( e ) LNCaP and U87 cells were infected with EV or MAN2C1 retrovirus, followed by selection with hygromycin for 3 days to achieve 100% transfection and then examined for AKT activation (AKT-P), AKT, ectopic MAN2C1 (using M2 anti-FLAG antibody) or actin by western blotting. Full size image α-MAN2C1 binds to PTEN To determine the underlying mechanism whereby MAN2C1 reduces PTEN function, we examined a possible interaction between MAN2C1 and PTEN. C-terminal FLAG-tagged MAN2C1 was expressed with or without PTEN in 293T cells. Immunoprecipitation (IP) of PTEN led to the recovery of MAN2C1 and vice versa , whereas a Ctrl IgG did not precipitate MAN2C1 and PTEN ( Fig. 2a ). Furthermore, endogenous MAN2C1 and PTEN also coimmunoprecipitated in DU145, MCF7 and NIH3T3 cells ( Fig. 2b ). Both MCF7 and NIH3T3 cells express higher levels of endogenous PTEN than DU145 cells ( Fig. 2b ), which likely correlate with the higher efficiencies of co-IP of endogenous PTEN via MAN2C1 ( Fig. 2b ). To further demonstrate the interaction between MAN2C1 and PTEN, we assessed their intracellular co-localization. Although endogenous MAN2C1 co-localized with endogenous PTEN in DU145 cells ( Fig. 2c ) and MCF7 cells ( Supplementary Fig. S2b ), their ectopic counterparts co-localized in LNCaP and 293T cells ( Supplementary Fig. S3 ). In addition, this co-localization was clearly demonstrated by three-dimentional reconstruction of a set of z -stack images ( Supplementary Movies 1 , 2 ). Taken together, we provide evidence demonstrating that MAN2C1 binds to and co-localizes with PTEN. 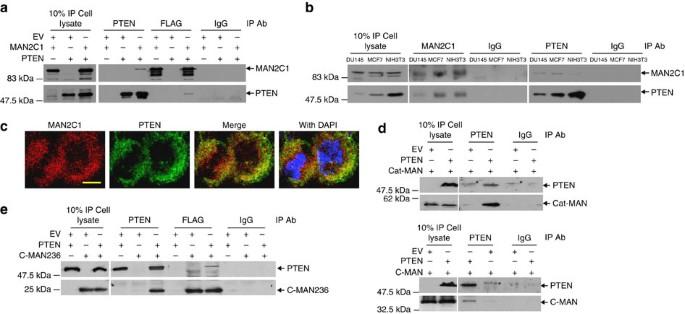Figure 2: MAN2C1 binds to and co-localizes with PTEN. (a) MAN2C1 and PTEN were expressed in 293T cells, followed by immunoprecipitation (IP) for PTEN, MAN2C1 (FLAG), or control (IgG), and western blot analysis for the indicated proteins. (b) IP and western blot analysis of endogenous MAN2C1 and PTEN in DU145, MCF7 and NIH3T3 cells. (c) A typicalz-stack image showing the co-localization between endogenous MAN2C1 (red) and PTEN (green) in DU145. Nuclei were counterstained with 4,6-diamidino-2-phenylindole (DAPI, blue). Scale bar, 10 μm. (d) Cat-MAN (top panel) or C-MAN (bottom panel) was coexpressed with PTEN in 293T cells, followed by coimmunoprecipitation of Cat-MAN (top panel) or C-MAN (bottom panel) with PTEN. *Indicates background bands. (e) Coimmunoprecipitation of the C-MAN236/PTEN complex with the indicated antibodies using the 293 cell-based transient expression system. Figure 2: MAN2C1 binds to and co-localizes with PTEN. ( a ) MAN2C1 and PTEN were expressed in 293T cells, followed by immunoprecipitation (IP) for PTEN, MAN2C1 (FLAG), or control (IgG), and western blot analysis for the indicated proteins. ( b ) IP and western blot analysis of endogenous MAN2C1 and PTEN in DU145, MCF7 and NIH3T3 cells. ( c ) A typical z -stack image showing the co-localization between endogenous MAN2C1 (red) and PTEN (green) in DU145. Nuclei were counterstained with 4,6-diamidino-2-phenylindole (DAPI, blue). Scale bar, 10 μm. ( d ) Cat-MAN (top panel) or C-MAN (bottom panel) was coexpressed with PTEN in 293T cells, followed by coimmunoprecipitation of Cat-MAN (top panel) or C-MAN (bottom panel) with PTEN. *Indicates background bands. ( e ) Coimmunoprecipitation of the C-MAN236/PTEN complex with the indicated antibodies using the 293 cell-based transient expression system. Full size image To characterize the putative binding domains in MAN2C1 that associate with PTEN, MAN2C1 truncation mutants were generated ( Supplementary Fig. S4a ). Both an amino (N)-terminal fragment encompassing the catalytic motif (Cat-MAN) and a C-terminal fragment of MAN2C1 (C-MAN) interacted with PTEN ( Fig. 2d ). Although the N-terminal 168 residues of C-MAN (C-MAN-N) did not bind to PTEN ( Supplementary Fig. S4b ), the C-terminal 236 residues of C-MAN (C-MAN236) interacted with PTEN ( Fig. 2e ). Further deletion of the N-terminal 103 residues from C-MAN236 (C-MAN236-C) greatly reduced its binding affinity to PTEN ( Supplementary Fig. S4c ). Collectively, these results demonstrate that MAN2C1 binds to PTEN by means of multiple domains, and that C-MAN236 is capable of PTEN interaction, consistent with our initial identification of the C-MAN236 fragment from our screen ( Supplementary Fig. S1a ). α-MAN2C1 inhibits the PIP 3 phosphatase activity of PTEN Our observations that MAN2C1 reduces PTEN function ( Fig. 1 ) and binds to PTEN ( Fig. 2 ) prompted us to determine whether MAN2C1 inhibits the PIP 3 phosphatase activity of PTEN. Recombinant glutathione S -transferase (GST)-PTEN and GST-MAN2C1 were purified using Escherichia coli ( Fig. 3a ) and their identities were confirmed by western blot ( Fig. 3a ). In comparison to GST, GST-MAN2C1 dose-dependently inhibited the PIP 3 phosphatase activity of GST-PTEN ( Fig. 3b ). To examine whether MAN2C1 inhibits cellular PTEN-mediated PIP 3 phosphatase activity, we transiently expressed the phosphatase-deficient PTEN(C124S), PTEN, MAN2C1 or PTEN+MAN2C1 in 293T cells ( Fig. 3c ). Although ectopic PTEN, immunoprecipitated by anti-HA antibody (Y-11), was competent to dephosphorylate PIP 3 in vitro , PTEN(C124S) displayed no such activity, as expected ( Fig. 3c ). MAN2C1 dose-dependently reduced PTEN-mediated PIP 3 phosphatase activity ( Fig. 3c ). At the ratio of 20:5 (MAN2C1:PTEN), MAN2C1 reduced the PIP 3 phosphatase activity to a level comparable to PTEN(C124S)-associated background activity ( Fig. 3c ), showing that MAN2C1 is able to completely inhibit the PIP 3 phosphatase activity of PTEN. 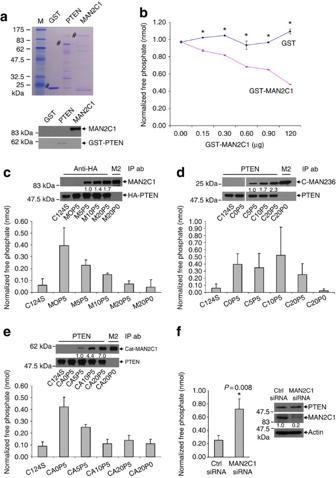Figure 3: MAN2C1 inhibits the PIP3phosphatase activity of PTEN. (a) The indicated recombinant GST fusion proteins (GST, GST-PTEN/PTEN and GST-MAN2C1/MAN2C1) were purified fromE. coliand 0.5 μg of individual recombinant proteins were analysed. #Indicates the molecular mass of the respective recombinant proteins (top panel). Western blotting was performed on 5 ng of individual recombinant proteins using anti-MAN2C1 or anti-PTEN antibodies (bottom panel). (b) The indicated doses of GST or GST-MAN2C1 were assayed for their effect on 0.3 μg GST-PTEN associated PIP3phosphatase activity. Experiments were repeated three times. Means±standard derivations are shown. *P<0.05 (two-tailed Student'st-test). (c–e) A quantity of 5 μg PTEN (P5) and 0, 5, 10 and 20 μg MAN2C1 (M0P5, M5P5, M10P5, M20P5) (c), C-MAN236 (C0P5, C5P5, C10P5, C20P5) (d) or Cat-MAN (CA0P5, CA5P5, CA10P5, CA20P5) (e) were coexpressed in 293T cells and IP with indicated antibody and 60 μl agarose G matrix. A volume of 15 μl matrix was used to perform the lipid phosphatase assay. 5 μg PTEN(C124S) (C124S) and 20 μg MAN2C1 (M20P0) (c), C-MAN236 (C20P0) (d) or Cat-MAN (CA20P0) (e) were expressed in 293T cells and IP accordingly. IP proteins were detected by western blotting. The assay was performed four times. Values are presented as mean±standard deviation. Coimmunoprecipitated MAN2C1 and its mutants (c–e) were quantified and presented as fold changes underneath the individual panels. (f) DU145 cells were transfected with control (Ctrl) or MAN2C1 siRNA lentivirus and selected in puromycin for 48 h to ensure 100% infection. Cells were then analysed for the expression of PTEN, MAN2C1 and actin (right panel). MAN2C1 levels were quantified and presented as fold changes in comparison with Ctrl siRNA cells underneath the individual panels. PTEN was IP from Ctrl and MAN2C1 siRNA-treated cells and assayedin vitrofor its PIP3phosphatase activity. Experiments were repeated three times and presented as means±standard deviations. Results were analysed by two-tailed Student'st-test. Figure 3: MAN2C1 inhibits the PIP 3 phosphatase activity of PTEN. ( a ) The indicated recombinant GST fusion proteins (GST, GST-PTEN/PTEN and GST-MAN2C1/MAN2C1) were purified from E. coli and 0.5 μg of individual recombinant proteins were analysed. #Indicates the molecular mass of the respective recombinant proteins (top panel). Western blotting was performed on 5 ng of individual recombinant proteins using anti-MAN2C1 or anti-PTEN antibodies (bottom panel). ( b ) The indicated doses of GST or GST-MAN2C1 were assayed for their effect on 0.3 μg GST-PTEN associated PIP 3 phosphatase activity. Experiments were repeated three times. Means±standard derivations are shown. * P <0.05 (two-tailed Student's t -test). ( c – e ) A quantity of 5 μg PTEN (P5) and 0, 5, 10 and 20 μg MAN2C1 (M0P5, M5P5, M10P5, M20P5) ( c ), C-MAN236 (C0P5, C5P5, C10P5, C20P5) ( d ) or Cat-MAN (CA0P5, CA5P5, CA10P5, CA20P5) ( e ) were coexpressed in 293T cells and IP with indicated antibody and 60 μl agarose G matrix. A volume of 15 μl matrix was used to perform the lipid phosphatase assay. 5 μg PTEN(C124S) (C124S) and 20 μg MAN2C1 (M20P0) ( c ), C-MAN236 (C20P0) ( d ) or Cat-MAN (CA20P0) ( e ) were expressed in 293T cells and IP accordingly. IP proteins were detected by western blotting. The assay was performed four times. Values are presented as mean±standard deviation. Coimmunoprecipitated MAN2C1 and its mutants ( c – e ) were quantified and presented as fold changes underneath the individual panels. ( f ) DU145 cells were transfected with control (Ctrl) or MAN2C1 siRNA lentivirus and selected in puromycin for 48 h to ensure 100% infection. Cells were then analysed for the expression of PTEN, MAN2C1 and actin (right panel). MAN2C1 levels were quantified and presented as fold changes in comparison with Ctrl siRNA cells underneath the individual panels. PTEN was IP from Ctrl and MAN2C1 siRNA-treated cells and assayed in vitro for its PIP 3 phosphatase activity. Experiments were repeated three times and presented as means±standard deviations. Results were analysed by two-tailed Student's t -test. Full size image As both Cat-MAN and C-MAN236 interact with PTEN ( Fig. 2d,e ), we transiently expressed PTEN(C124), PTEN, PTEN+Cat-MAN or PTEN+C-MAN236 in 293T cells. IP of PTEN dose-dependently precipitated C-MAN236 and Cat-MAN, respectively ( Fig. 3d,e ). In comparison with the negative PTEN(C124S) and positive PTEN Ctrls, Cat-MAN ( Fig. 3e ), but not C-MAN236 ( Fig. 3d ), dose-dependently inhibited the PIP 3 phosphatase activity of PTEN. To confirm these findings, we directly analysed endogenous PTEN-mediated PIP 3 phosphatase activity following knockdown of MAN2C1. In comparison to Ctrl siRNA treatment, MAN2C1 siRNA significantly reduced MAN2C1 protein and enhanced the PIP 3 phosphatase activity of PTEN in DU145 cells ( Fig. 3f ). To further confirm the physiological relevance of MAN2C1 in inhibiting PTEN activity, we have knocked down MAN2C1 in immortalized but non-transformed human prostate epithelial BPH-1 cells [39] , [40] , [41] ( Fig. 4a ). Knockdown of PTEN enhanced AKT activation, as expected ( Fig. 4a ). Knockdown of MAN2C1 reduced ATK activation ( Fig. 4a ). This depended on the existence of endogenous PTEN, as concomitant knockdown of PTEN rendered MAN2C1 siRNA ineffective in inhibiting AKT activation ( Fig. 4a ), indicating that knockdown of MAN2C1 leads to an increase in PTEN-derived PIP 3 phosphatase activity. Indeed, knockdown of MAN2C1 increased the PIP 3 phosphatase activity of endogenous PTEN ( Fig. 4b ). Furthermore, knockdown of MAN2C1 also elevated endogenous PTEN-mediated PIP 3 phosphatase activity in primary human prostate epithelial cells ( Fig. 4c ). 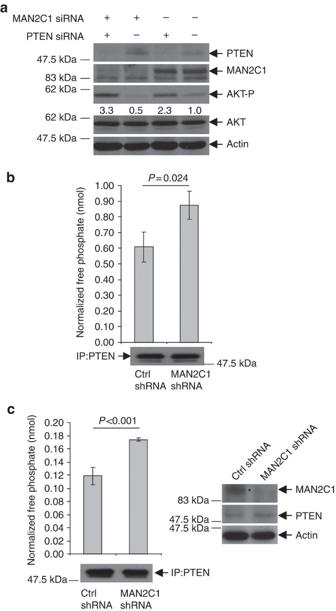Figure 4: MAN2C1 inhibits PTEN-derived PIP3phosphatase activity in both immortalized and primary human prostate epithelial cells. (a) Immortalized human prostate epithelial BPH-1 cells were infected with MAN2C1 shRNA, PTEN shRNA, their combination, or control shRNA (−) lentivirus as indicated, followed by western blot analysis for PTEN, MAN2C1, phosphorylation of AKT S473 (AKT-P), total AKT and actin. The levels of AKT-P were quantified against AKT and presented under the AKT-P panel as fold changes in comparison with mock-treated cells. (b) PTEN was immunoprecipitated from Ctrl (control) shRNA and MAN2C1 shRNA lentivirus-infected cells (IP:PTEN) and then assayed for PTEN-dependent PIP3phosphatase activityin vitro. Experiments were repeated three times and presented as mean±standard deviation. Results were analysed by two-tailed Student'st-test. (c) Human primary epithelial cells were purchased from Sciencell Research labs and infected with a Ctrl shRNA or MAN2C1 shRNA lentivirus. The expression of MAN2C1 (*MAN2C1 band), PTEN and actin was examined by western blot (right panel). PTEN-dependent PIP3phosphatase activity was then determined following immunoprecipitation of PTEN (IP:PTEN). Experiments were repeated three times and presented as mean±standard deviation. Results were analysed by two-tailed Student'st-test. Figure 4: MAN2C1 inhibits PTEN-derived PIP 3 phosphatase activity in both immortalized and primary human prostate epithelial cells. ( a ) Immortalized human prostate epithelial BPH-1 cells were infected with MAN2C1 shRNA, PTEN shRNA, their combination, or control shRNA (−) lentivirus as indicated, followed by western blot analysis for PTEN, MAN2C1, phosphorylation of AKT S473 (AKT-P), total AKT and actin. The levels of AKT-P were quantified against AKT and presented under the AKT-P panel as fold changes in comparison with mock-treated cells. ( b ) PTEN was immunoprecipitated from Ctrl (control) shRNA and MAN2C1 shRNA lentivirus-infected cells (IP:PTEN) and then assayed for PTEN-dependent PIP 3 phosphatase activity in vitro . Experiments were repeated three times and presented as mean±standard deviation. Results were analysed by two-tailed Student's t -test. ( c ) Human primary epithelial cells were purchased from Sciencell Research labs and infected with a Ctrl shRNA or MAN2C1 shRNA lentivirus. The expression of MAN2C1 (*MAN2C1 band), PTEN and actin was examined by western blot (right panel). PTEN-dependent PIP 3 phosphatase activity was then determined following immunoprecipitation of PTEN (IP:PTEN). Experiments were repeated three times and presented as mean±standard deviation. Results were analysed by two-tailed Student's t -test. Full size image α-MAN2C1 promotes tumourigenesis by inhibiting PTEN Our observations that MAN2C1 inhibits PTEN-dependent PIP 3 phosphatase activity and enhances the activities of the PI3K-AKT pathway, strongly suggest that MAN2C1 could promote tumourigenesis. To investigate this possibility, we examined whether MAN2C1 enhances the ability of DU145 cells to form xenograft tumours in immunocompromised mice. By taking advantage of the fact that DU145 cells form xenograft tumours inefficiently in nude mice (He and Tang, unpublished observation), we subcutaneously (s.c.) implanted DU145 EV cells and DU145 MAN2C1 overexpressing cells into these animals. Although DU145 EV cells formed small tumours with low efficiency, DU145 cells expressing MAN2C1 formed significantly larger xenograft tumours ( Fig. 5a , Table 1 , Supplementary Fig. S5a ). These xenografted tumours, as expected, expressed ectopic MAN2C1 and endogenous PTEN with elevated AKT activation ( Supplementary Fig. S5b ). 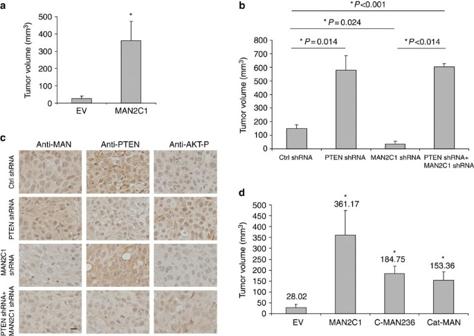Figure 5: MAN2C1 promotes the formation of DU145 cell-derived xenograft tumours by inactivating PTEN. (a) EV and MAN2C1 expressing DU145 cells (5×106) were implanted into flanks of NU/NU mice. Five mice were used for each treatment and animals were terminated at 38 days. Tumour volumes are presented as means±standard derivations. (b) DU145 cells were infected with retrovirus expressing shRNA for MAN2C1, PTEN or both, and then cultured in the presence of puromycin (for MAN2C1 shRNA retrovirus), hygromycin (for PTEN shRNA retrovirus) or both for 2–3 days to achieve 100% infection. A total of 2×105cells were subsequently implanted into NOD/SCID mice and the mice were killed after 8 weeks. Tumour volumes are presented as means±standard derivations. The asterisk indicates statistical significance (two-tailed Student'st-test) for indicated comparisons,P=0.014 for Ctrl shRNA versus PTEN shRNA,P=0.024 for Ctrl shRNA versus MAN2C1 shRNA,P<0.001 for both Ctrl shRNA versus PTEN shRNA/MAN2C1 shRNA and MAN2C1 shRNA versus MAN2C1/PTEN shRNAs. (c) Representative immunohistochemistry to demonstrate MAN2C1, PTEN and AKT-P expression in tumours derived from each of the cell lines inb. Scale bar, 10 μm. (d) DU145 cells were transfected with an empty retrovirus (EV) or retrovirus expressing MAN2C1, C-MAN236 or Cat-MAN, followed by selection of cells with hygromycin for 2 days to ensure 100% transfection. Five nude mice were s.c. injected with 5×106of the respective cells. Tumour volumes are presented as means±standard derivations. The asterisk representsP<0.05 for all transgene-derived xenograft tumours versus EV xenograft tumours and MAN2C1 tumours versus the tumours of C-MAN236 and Cat-MAN. All statistical analysis was performed using two-tailed Student'st-test. Figure 5: MAN2C1 promotes the formation of DU145 cell-derived xenograft tumours by inactivating PTEN. ( a ) EV and MAN2C1 expressing DU145 cells (5×10 6 ) were implanted into flanks of NU/NU mice. Five mice were used for each treatment and animals were terminated at 38 days. Tumour volumes are presented as means±standard derivations. ( b ) DU145 cells were infected with retrovirus expressing shRNA for MAN2C1, PTEN or both, and then cultured in the presence of puromycin (for MAN2C1 shRNA retrovirus), hygromycin (for PTEN shRNA retrovirus) or both for 2–3 days to achieve 100% infection. A total of 2×10 5 cells were subsequently implanted into NOD/SCID mice and the mice were killed after 8 weeks. Tumour volumes are presented as means±standard derivations. The asterisk indicates statistical significance (two-tailed Student's t -test) for indicated comparisons, P =0.014 for Ctrl shRNA versus PTEN shRNA, P =0.024 for Ctrl shRNA versus MAN2C1 shRNA, P <0.001 for both Ctrl shRNA versus PTEN shRNA/MAN2C1 shRNA and MAN2C1 shRNA versus MAN2C1/PTEN shRNAs. ( c ) Representative immunohistochemistry to demonstrate MAN2C1, PTEN and AKT-P expression in tumours derived from each of the cell lines in b . Scale bar, 10 μm. ( d ) DU145 cells were transfected with an empty retrovirus (EV) or retrovirus expressing MAN2C1, C-MAN236 or Cat-MAN, followed by selection of cells with hygromycin for 2 days to ensure 100% transfection. Five nude mice were s.c. injected with 5×10 6 of the respective cells. Tumour volumes are presented as means±standard derivations. The asterisk represents P <0.05 for all transgene-derived xenograft tumours versus EV xenograft tumours and MAN2C1 tumours versus the tumours of C-MAN236 and Cat-MAN. All statistical analysis was performed using two-tailed Student's t -test. Full size image Table 1 Tumourigenicity of DU145 and its derivative cells. Full size table We subsequently determined the role of endogenous MAN2C1 in inhibiting endogenous PTEN function during tumourigenesis. As reported previously [32] , [42] , we used a transient knockdown system and nonobese diabetes/severe combined immunodeficiency (NOD/SCID) mice were used, as this host produces xenograft tumours with a higher efficiency than nude mice (He and Tang, unpublished observation). DU145 cells were transiently treated with a combination of Ctrl siRNA, MAN2C1 siRNA and/or PTEN siRNA oligonucleotides before being s.c. implanted into NOD/SCID mice. Although knockdown of PTEN seems to facilitate tumour formation at early stages compared with Ctrl siRNA tumours ( Table 1 , see the tumour volumes for Ctrl siRNA and PTEN siRNA treatments at 21 and 28 days after implantation), both PTEN siRNA-treated cells and Ctrl siRNA-treated cells formed tumours with a comparable efficiency at later stages ( Table 1 ). This might be attributable to the transient nature of siRNA treatment. Knockdown of MAN2C1, however, significantly reduced the rate of tumour formation, which was largely reversed when PTEN was concomitantly knocked down ( Table 1 , Supplementary Fig. S5c ). To confirm these observations and also to overcome the shortcomings associated with the transient knockdown of PTEN and MAN2C1, we stably knocked down PTEN and MAN2C1 individually, and in combination. Xenograft tumours were then generated using these lines. Tumour incidence was 5/5 for all groups except for MAN2C1 knockdown cells, in which 3/5 implantations formed small tumours. As expected, knockdown of PTEN significantly enhanced DU145 cell-derived xenograft tumours ( Fig. 5b ). Knockdown of MAN2C1 significantly reduced the formation of xenograft tumours, which was reversed by concomitant knockdown of PTEN ( Fig. 5b ). In addition, knockdown of individual proteins was not only confirmed by immunohistochemistry (IHC) in the respective xenograft tumours, but it was also observed that knockdown of MAN2C1 reduced AKT activation (AKT S473 phosphorylation) in a PTEN-dependent manner ( Fig. 5c ); that is, knockdown of MAN2C1 was incapable of reducing AKT activation when PTEN was co-knocked down ( Fig. 5c ). This result, thus, demonstrates that MAN2C1 promotes the formation of DU145 cell-derived xenograft tumours, at least in part, by inhibiting endogenous PTEN function. α-MAN2C1-mediated tumourigenesis by inhibiting PTEN Although both Cat-MAN and C-MAN236 bind PTEN ( Fig. 2d,e ), only Cat-MAN inhibits the PIP 3 phosphatase activity of PTEN ( Fig. 3d,e ). We thus examined how Cat-MAN and C-MAN236 affect tumourigenesis. In comparison with EV, both fragments, when ectopically expressed in DU145 cells, promote xenograft tumour formation ( Fig. 5d ). Although inhibiting the PIP 3 phosphatase activity of PTEN likely contributes to Cat-MAN-mediated tumourigenic activity, C-MAN236 may promote xenograft tumour formation by inhibiting other regulatory events that affect PTEN function, including recruitment of PTEN to the plasma membrane. This concept is supported by the observation that ectopic C-MAN236 co-localizes with endogenous PTEN in DU145 cells ( Supplementary Fig. S6a ). Consistent with MAN2C1 being an ER protein [33] , ectopic C-MAN236 largely co-localizes with KDEL (a C-terminal ER retention sequence present in several ER-resident chaperones [43] ) in DU145 cells ( Supplementary Fig. S6a ). C-MAN236 cofractionated with calnexin-containing ER microsomes ( Supplementary Fig. S6b ), further supporting its ER localization. More importantly, although ectopic PTEN failed to associate with microsomes, 28% of ectopic PTEN cofractionated with microsomes following C-MAN236 co-transfection ( Supplementary Fig. S6b ). Furthermore, ∼ 31% of endogenous PTEN co-localized with the ER-resident chaperone GRP78 in DU145 cells, with C-MAN236 expression increasing this co-localization to 64.7% (determined by analysis of the confocal images using IMARIS software). The concept that Cat-MAN and C-MAN236 may promote tumourigenesis by inhibiting different aspects of PTEN regulation is consistent with the observation that MAN2C1 is more potent than either Cat-MAN or C-MAN236 in promoting the formation of DU145 cell-derived xenograft tumours ( Fig. 5d ). α-MAN2C1 associates with reduction of PTEN function Approximately 50% of PCs display normal PTEN expression [17] . Given that MAN2C1 inhibits PTEN function and promotes DU145 PC cells forming tumours in mice by suppressing PTEN function, we investigated the possibility that MAN2C1 associates with attenuation of PTEN function in PTEN-positive primary PCs. Consistent with the co-localization of PTEN with MAN2C1 in DU145 PC cells, we were able to detect in our collection of PC tissues ( Supplementary Table S2 ) that PTEN co-localizes with MAN2C1 in PTEN-positive prostate tumour cells ( Fig. 6a ). Interestingly, in PTEN-negative carcinomas, MAN2C1 expression was also low ( Fig. 6a ). The differences in PTEN and MAN2C1 staining between PTEN-positive and PTEN-negative carcinomas did not result from variations in immunofluorescent staining, as these carcinomas were from the same specimen ( Fig. 6a ). 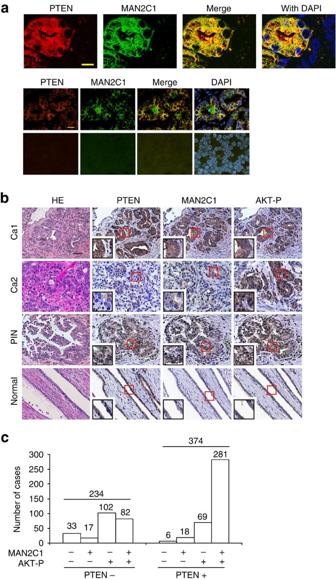Figure 6: Correlation of MAN2C1 expression with loss of PTEN function in primary prostate cancer. (a) Representative images of dual-IF (immunofluorescent) staining of prostate cancer tissues for PTEN (red) or MAN2C1 (green). Nuclei were counterstained with 4,6-diamidino-2-phenylindole (DAPI, blue). PTEN-positive (upper two panels) and -negative (lower panel) carcinomas in the same patient are shown. Scale bar represents 10 and 25 μm, respectively. Images were captured using a Zeiss LSM510 confocal microscrope and LSM510 Control Imaging software. (b) Hematoxylin and eosin (HE) and IHC staining of carcinoma (Ca), high-grade PIN and normal prostatic gland. All tissues were from the same patient/slide. Scale bar, 50 μm. (c) TMA2+TMA5 were IHC stained and analysed as a pooled population. Scores were grouped as negative (0) or positive (1). The number of cases expressing MAN2C1 (+ or −), AKT-P (+ or −) and PTEN (+ or −) are indicated on the top of individual bars. Figure 6: Correlation of MAN2C1 expression with loss of PTEN function in primary prostate cancer. ( a ) Representative images of dual-IF (immunofluorescent) staining of prostate cancer tissues for PTEN (red) or MAN2C1 (green). Nuclei were counterstained with 4,6-diamidino-2-phenylindole (DAPI, blue). PTEN-positive (upper two panels) and -negative (lower panel) carcinomas in the same patient are shown. Scale bar represents 10 and 25 μm, respectively. Images were captured using a Zeiss LSM510 confocal microscrope and LSM510 Control Imaging software. ( b ) Hematoxylin and eosin (HE) and IHC staining of carcinoma (Ca), high-grade PIN and normal prostatic gland. All tissues were from the same patient/slide. Scale bar, 50 μm. ( c ) TMA2+TMA5 were IHC stained and analysed as a pooled population. Scores were grouped as negative (0) or positive (1). The number of cases expressing MAN2C1 (+ or −), AKT-P (+ or −) and PTEN (+ or −) are indicated on the top of individual bars. Full size image To examine whether this co-localization presaged a reduction in PTEN function, we determined the expression of PTEN, MAN2C1 and AKT activation (AKT-P) by IHC in normal prostate glands, PINs (prostatic intraepithelial neoplasia) and carcinomas within the same primary tissues/slides. Immunodetection of PTEN, MAN2C1 and AKT-P was observed in normal prostate gland, PINs and carcinoma ( Fig. 6b ). However, the levels of AKT-P in normal prostatic glands were much lower than those present in PINs and carcinomas ( Fig. 6b ). The staining was specific as Ctrl IgG did not reveal detectable signal, anti-MAN2C1 antibody specifically recognized MAN2C1 by IHC ( Supplementary Fig. S7 ); and in the majority of PTEN-negative carcinomas, anti-MAN2C1 antibody did not produce detectable signals ( Fig. 6a,b ). Both PTEN-positive and -negative carcinomas showed increased AKT-P, but only PTEN-positive carcinomas displayed intense MAN2C1 staining together with enhanced AKT activation ( Fig. 6b ). This phenomenon was generally observed in our IHC study, which demonstrates MAN2C1 upregulation in PTEN-positive PCs as well as attenuation of PTEN function in these PCs (see later sections for details). To confirm this correlation, in addition to our patient cohort ( Supplementary Table S2 ), we examined by IHC two independent patient cohorts, tissue microarrays 2 and 5 (TMA2, TMA5; Supplementary Data 1 and 2 ). IHC staining of 608 (234+374) ( Fig. 6c ) patients in the pooled patient cohort (TMA2+5) revealed that 38.5% (234/608) of carcinomas were PTEN negative, in which 42.3% (99(17+82)/234) were MAN2C1 positive ( Fig. 6c ); 61.5% (374/608) of carcinoma are PTEN positive, in which 79.9% (299(18+281)/374) were MAN2C1 positive ( Fig. 6c ); 78.6% (184(102+82)/234) of PTEN-negative carcinomas displayed AKT activation (AKT-P), in which 44.6% (82/184(102+82)) were MAN2C1 positive ( Fig. 6c ); and of the PTEN-positive carcinomas, 93.6% (350(69+281)/374) exhibited intensive AKT-P staining ( Fig. 6c ), in which 80.3% (281/350(69+281)) showed intensive MAN2C1 staining ( Fig. 6c ). Similar observations were also obtained in carcinomas and in PINs in the individual patient cohorts ( Supplementary Tables S3–S5 ). MAN2C1 positively correlated with PTEN expression (Pearson Correlation Coefficient: Pearson's ϕ: 0.385, P <0.001 determined by χ 2 test) and AKT activation in prostate carcinomas (Pearson's ϕ: 0.142, P <0.001). PTEN also positively correlated with AKT activation in prostate carcinomas (Pearson's ϕ: 0.222, P <0.001). These correlations were also observed in PINs and carcinomas in individual patient cohorts ( Supplementary Tables S3–S5 ) but not in normal prostate glands ( Supplementary Tables S3, S5 ). Upregulation of α-MAN2C1 in PTEN-positive PC On the basis of the above observations that MAN2C1 associates with attenuation of PTEN function and that low levels of MAN2C1 were observed in PTEN-negative PCs ( Fig. 6 ), we reasoned that MAN2C1 might be specifically upregulated in PTEN-positive primary PCs. To address this issue, we determined MAN2C1 expression in PTEN-positive versus PTEN-negative primary prostate carcinomas. The results showed that MAN2C1 expression increased significantly only in PTEN-positive PINs and carcinomas in the presence of AKT activation, but not in the PTEN-negative counterparts ( Fig. 7a , Supplementary Table S6 ). In addition, MAN2C1 expression significantly increases only in PTEN-positive PINs and carcinomas of all Gleason scores (except Gleason 5, which might be due to insufficient patient numbers), but not in the PTEN-negative counterparts in TMA2+TMA5 ( Supplementary Fig. S8 , Supplementary Table S7 ). There was no difference in MAN2C1 expression between PIN and carcinomas of different Gleason scores. 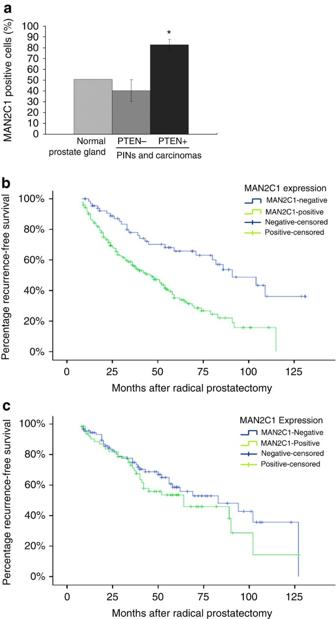Figure 7: The association of MAN2C1 with the biochemical recurrence of PTEN-positive prostate cancer. (a) The percentages of MAN2C1-positive cells in normal prostate glands, as well as in PTEN-positive and -negative PINs and carcinomas, were determined on the basis of the IHC staining of TMA2 and TMA 5. Results were derived from four biological replicates. Means±standard derivations are shown. *P<0.05 (two-tailed Student'st-test) in comparison with PTEN-negative PINs and carcinomas. (b,c) MAN2C1 associates with biochemical recurrence, defined as rising serum levels of prostate-specific antigen (PSA) after radical prostatectomy, in PTEN-positive prostate cancer. Kaplan–Meier analysis of biochemical recurrence-free survival for a subset of PTEN-positive PC patients (b,n=240; log-rank test statistic=18.137,P<0.01) and PTEN-negative PC patients (c,n=153; log-rank test statistic=0.307,P=0.307) with MAN2C1-positive or MAN2C1-negative PC. Data were generated using TMA5. Censored patients in MAN2C1-negative (negative-censored) and MAN2C1-positive (positive-censored) populations are indicated. Figure 7: The association of MAN2C1 with the biochemical recurrence of PTEN-positive prostate cancer. ( a ) The percentages of MAN2C1-positive cells in normal prostate glands, as well as in PTEN-positive and -negative PINs and carcinomas, were determined on the basis of the IHC staining of TMA2 and TMA 5. Results were derived from four biological replicates. Means±standard derivations are shown. * P <0.05 (two-tailed Student's t -test) in comparison with PTEN-negative PINs and carcinomas. ( b , c ) MAN2C1 associates with biochemical recurrence, defined as rising serum levels of prostate-specific antigen (PSA) after radical prostatectomy, in PTEN-positive prostate cancer. Kaplan–Meier analysis of biochemical recurrence-free survival for a subset of PTEN-positive PC patients ( b , n =240; log-rank test statistic=18.137, P <0.01) and PTEN-negative PC patients ( c , n =153; log-rank test statistic=0.307, P =0.307) with MAN2C1-positive or MAN2C1-negative PC. Data were generated using TMA5. Censored patients in MAN2C1-negative (negative-censored) and MAN2C1-positive (positive-censored) populations are indicated. Full size image α-MAN2C1 associates with PC recurrence Recurrent cancer is the leading cause of cancer-associated deaths. In an effort to address whether MAN2C1 expression associates with PC recurrence, we observed that in TMA5, which was organized according to PC recurrence (see Methods for details), Kaplan–Meier survival analysis revealed that patients with MAN2C1-positive PC were significantly associated with decreased recurrence-free survival ( Fig. 7b ). Similar observations were also obtained in our patient cohort and TMA2, although with less number of patients ( Supplementary Fig. S9 ). As MAN2C1 was also detected in a small proportion of PTEN-negative carcinomas ( Fig. 6c ), we further determined the groups of patients (PTEN-positive versus PTEN-negative) in which MAN2C1 associates with PC recurrence. Interestingly, MAN2C1 associates with decreased recurrence-free survival only in patients displaying PTEN-positive PC ( Fig. 7b,c ). Taken together, these observations support the concept that MAN2C1 mediates PTEN inactivation in PC cells. Genetic alternations in the PTEN gene are frequently detected in a variety of human cancers [4] . Although PTEN is infrequently mutated in sporadic colorectal cancers, ∼ 19% of those cancers with high levels of microsatellite instability have the PTEN promoter hypermethylated [16] . Reduction of the PTEN protein without mutations in the PTEN gene has been observed in PC [17] . Besides these genetic and/or epigenetic events that lead to loss of PTEN function, putative PTEN-NRs may also attenuate PTEN function during the process of tumourigenesis. This possibility is supported by recent reports that PTEN is expressed normally but with impaired function in human cancers [28] , [29] . Although the function PTEN can be indirectly inhibited by factors including DJ-1 and Surivin [44] , [45] , P-REX2a and SIPL1 have been reported to inhibit PTEN by binding to PTEN during breast and cervical tumourigenesis [31] , [32] . It is therefore possible that different NRs of PTEN may inhibit PTEN by binding to PTEN in different types of human cancers. In this study, we identified MAN2C1 as a NR of PTEN in PC cells. The α-mannosidase family is involved in glycoprotein maturation in the ER and Golgi [34] . Although MAN2C1 has been suggested to have a role in the aforementioned process, it remains to be determined whether the catalytic activity of MAN2C1 contributes to PTEN inactivation. Our observation that MAN2C1 associates with prostate tumourigenesis is consistent with reports that overexpression of MAN2C1 transforms human B cells [35] and that reduction in MAN2C1 suppresses the metastasis of nasopharyngeal carcinoma [36] . Interestingly, MAN2C1 transgenic mice that have recently been developed are prone to enhanced tumour growth, invasion and metastasis [46] . These investigators speculated that the mechanism might be through impaired antibody response to tumour antigens, but this was not specifically studied. Mechanistically, MAN2C1 promotes the formation of DU145 cell-derived xenograft tumours at least in part by inhibiting the PIP 3 phosphatase activity of PTEN by binding to PTEN. However, this may not be the only mechanism responsible for MAN2C1 to inhibit PTEN function, as C-MAN236 also attenuates PTEN function without inhibiting the PIP 3 phosphatase activity of PTEN. Although C-MAN236 does not inhibit PTEN-derived PIP 3 phosphatase activity, it may impair PTEN function by reducing the plasma membrane recruitment of PTEN by binding to PTEN ( Supplementary Fig. S6 ). This concept is consistent with MAN2C1 being an ER protein [33] . In addition, both MAN2C1 and C-MAN236 are exclusively ER proteins when overexpressed in DU145 and other cells. This possibility is also in line with the observation that ectopic PTEN associates with the ER in C-MAN236 overexpressing cells ( Supplementary Fig. S6 ). In addition, a similar mechanism was reported, in which caspase 7 was recruited to ER through interaction with GRP78, leading to prevention of its apoptotic activity in response to etoposide [47] . It is also possible that the catalytic activity of MAN2C1 may also contribute to the inactivation of PTEN at the ER. This may be achieved by MAN2C1-mediated alteration of glycosylation on specific components of the MAN2C1/PTEN complex, which may result in reduction of PTEN function. On the other hand, it remains an intriguing possibility that PTEN may in turn affect the mannose-trimming activity of MAN2C1 towards its substrates. As changes in the patterns of protein glycosylation are well known to associate with oncogenesis [48] , PTEN may regulate this aspect of tumourigenesis by potentially regulating MAN2C1 function. As MAN2C1 has been demonstrated to hydrolyse p -nitrophenyl-α- D -mannopyranoside [33] , the notion whether PTEN may influence the enzymatic activity of MAN2C1 can thus be readily tested. The PI3K pathway has essential roles in tumourigenesis by coordination of cell cycle progression, survival and cytoskeletal organization [5] . PTEN is the major mechanism that suppresses the PI3K pathway, as loss of PTEN activates the PI3K-AKT pathway in mice and in cells [19] , [49] , [50] , [51] . Therefore, attenuation of PTEN function represents a major step during tumourigenesis. Although the PTEN gene is frequently mutated in human cancers [4] , [12] , a large population of breast and PCs express PTEN at physiological levels with elevated AKT activation [52] and high levels of PTEN and AKT activation were observed in renal cell carcinomas [28] . These observations suggest that PTEN is inactivated during tumourigenesis by its negative regulatory mechanisms in addition to the observed genetic and epigenetic events. We provide evidence that MAN2C1 is a novel PTEN-NR in PC cells. The possibility that MAN2C1 may also have a role in attenuation of PTEN function during the tumourigenesis of other types of PTEN-positive human cancers remains to be explored. Cell lines and retrovirus infection DU145, PC3, LNCaP, 293T, MCF7 and NIH3T3 lines were obtained from American Type Culture Collection and cultured according to the conditions specified. Immortalized human prostate epithelial BPH-1 cells were kindly provided by Dr Simon Hayward at Vanderbilt University Medical Center, Nashville, Tennessee, USA. Human primary prostate epithelial cells were purchased from Sciencell Research labs. At passage 2, human primary prostate epithelial cells were infected with a Ctrl or MAN2C1 siRNA lentivirus (Santa Cruz), selected in puromycin at 1 μg ml −1 for 36 h, and then analysed for protein expression and assayed for PTEN-derived PIP 3 phosphatase activity. Retrovirus infection was performed as described previously [53] . Collecting primary prostate cancer tissue Prostate tissue was collected at St Joseph's Hospital in Hamilton, Ontario, Canada under the approval from the local Ethics Board and consent from patients. Cancers were examined and graded by pathologists of the Hospital. Immunofluorescence and confocal microscopy Double immunofluorescence staining was carried out using the following antibodies: monoclonal anti-PTEN (A2B1, Santa Cruz, 1 μg ml −1 ) or a polyclonal anti-PTEN (1:100; Upstate Technologies), and polyclonal anti-FLAG or a monoclonal anti-FLAG (M2, 1:500; Sigma). FITC-Donkey anti-mouse IgG (1:200; Jackson Immuno Research), Rhodamine-Donkey anti-rabbit IgG (1:200; Jackson Immuno Research) and FITC-Goat anti-mouse IgM (1:200; Jackson Immuno Research) were used as secondary antibodies. For dual immunofluorescence staining, tissues were deparaffinized, rehydrated and subjected to antigen retrieval and endogenous peroxidase quenching as indicated for IHC. Tissue sections were blocked for 1 h at room temperature in 3% donkey serum and 3% BSA in TBST. Dual immunofluorescent staining was carried out using a TSA Plus kit (PerkinElmer) according to the manufacturer's protocol. Sections were counterstained with 4,6-diamidino-2-phenylindole. Images, including confocal, were captured using a MP Leica TCS SP5 confocal microscope (Leica). Images were analysed using IMARIS 6.2 and processed using CorelDraw 12 and Adobe Photoshop 7. Xenograft tumour formation The designed DU145 cells were resuspended in Minimum Essential Medium (MEM)/Matrigel mixture (1:1 volume), followed by implantation of 0.1 ml of this mixture s.c. into flanks of 8-week-old male nude or NOD/SCID mice (The Jackson Laboratory). Tumour volume was determined using the standard formula: L × W 2 ×0.52, where L and W are the longest and shortest diameters, respectively. The presence of each tumour nodule was confirmed by necropsy. All animal work was carried out according to experimental protocols approved by the McMaster University Animal Research Ethics Board. Western blot and immunoprecipitation Frozen PC tissue and the corresponding normal tissue from nine patients were crushed under liquid nitrogen and suspended on ice in lysis buffer containing 20 mM Tris (pH 7.4), 150 mM NaCl, 1 mM EDTA, 1 mM EGTA, 1% Triton X-100, 25 mM sodium pyrophosphate, 1 mM NaF, 1 mM β-glycerophosphate, 0.1 mM sodium orthovanadate, 1 mM PMSF, 2 μg ml −1 leupeptin and 10 μg ml −1 aprotinin. Cell lysates were prepared and western blot was performed according to our published procedure [53] . Cell lysates containing 200 μg of protein were incubated with specific antibodies plus Protein G agarose (Invitrogen) at 4 °C overnight and were then washed six times in a buffer containing 50 mM Tris (PH 7.5), 100 mM NaCl, 1.5 mM EGTA and 0.1% Triton X-100. Antibodies used for IP were monoclonal anti-PTEN (A2B1, Santa Cruz, 1 μg), monoclonal anti-HA (12CA5, Y-11, Santa Cruz, 1 μg), monoclonal anti-FLAG (M2, Sigma, 1 μg) for MAN2C1 and mouse IgG (Sigma, 1 μg) as a negative Ctrl. The IP was analysed by western blot using polyclonal anti-PTEN (Upstate, 1:100) and anti-FLAG (Sigma, 1:500). RNA interference PTEN siRNA was expressed by a retroviral-based H1 promoter-driven shRNA vector (pRIH). The PTEN targeting sequence was previously described in ref. 54 . PTEN was also knocked down by oligonucleotide PTEN siRNA (see Supplementary Table S1 for targeting sequences). The oligonucleotide MAN2C1 siRNA (Invitrogen) target sequence was as follows: 5′-ATAGCTGGTCTTCTCACCCTCTTTC-3′. MAN2C1 siRNA was transfected into cells, using Lipofectamine 2000 (Invitrogen) according to the manufacturer's protocol. We also performed a large-scale knockdown of MAN2C1 using a lentivirus system in DU145 PC cells, immortalized human prostate epithelial BPH-1 cells and human primary prostate epithelial cells to assay its effect on the PIP 3 phosphatase activity of PTEN. Briefly, a MAN2C1 siRNA lentiviral vector (MAN2C1 shRNA; a TAT-independent lentiviral vector) was purchased from Santa Cruz. This vector expresses a pool of MAN2C1 siRNA. Packaging plasmids were gifts from Dr Bryan E. Strauss (University of Sao Paulo School of Medicine, Brazil). MAN2C1 siRNA lentivirus was packaged according to a published methodology [55] . The PTEN siRNA retrovirus (PTEN shRNA) has been described in ref. 32 . PTEN lipid phosphatase assay PTEN with MAN2C1 was co-transfected into 293T cells. Ectopic PTEN was immunoprecipitated with an anti-PTEN antibody (A2B1, Santa Cruz, 1 μg) and subsequently assessed for phosphatase activity. Phosphatase assay was performed by the addition of 50-nM water-soluble DiC 8 -PtdIns(3,4,5)P 3 (Echelon) as a substrate to assay for immunoprecipitated PTEN and recombinant PTEN-derived PIP 3 phosphatase activity at 37 °C for 40 min. Released free phosphates were measured with BIOMOL Green reagent (BIOMOL) and were normalized against a reaction containing PIP 3 substrate only [56] . Immunohistochemistry Paraffin-embedded sections of PC specimens were deparaffinized and heat-treated for 20 min in a 10 mM sodium citrate buffer (pH 6.0) in a food steamer. The following primary antibodies were incubated with the sections overnight at 4 °C: anti-MAN2C1 (1:500), anti-PTEN (1:100, A2B1, Santa Cruz) and anti-Ser473 phosphorylated AKT (1:200, Cell Signalling). Biotinylated goat anti-rabbit IgG (1:200) and avidin–biotin complex (ABC) were then added (Vectastain ABC kit, Vector Laboratories). Chromogen reaction was carried out with diaminobenzidine, and counterstaining was done with hematoxylin. An average staining score was given to representative sections from each sample. The intensity of staining was graded on a scale of 1–3, where 1 (low)=less than 20% of cells stained, 2 (medium)= 20–60% of the cells were stained and 3 (high)= >60% of cells were stained. For statistical analysis, scores 0–1 and 2–3 were grouped as 0 and 1, respectively, which were analysed using SPSS 10.0 software. Pearson's ϕ coefficient (Pearson's r computed on two dichotomous variables) was used to test for correlation between MAN2C1 and PTEN, and MAN2C1 and AKT pSer473 in normal, PIN and carcinoma. All tests were two tailed. A P -value <0.05 was considered statistically significant. Recurrence-free survival analysis Kaplan–Meier survival analysis was performed for a subset of 20 patients, obtained from the patients in our hospital, who had follow-up data following radical prostatectomy of at least 5 years (mean age±s.d.=62.3±7.0 years, range=50–72 years; mean Gleason score±s.d.=6.8±0.8, range=6–8; mean preoperative prostate-specific antigen (PSA)±s.d.=11.3±9.9 ng ml −1 ; range=2.6–40.5 ng ml −1 ). Median follow-up time was 69.5 months. Biochemical recurrence (first documented increase in serum PSA levels >0.2 ng ml −1 after radical prostatectomy) was used as the endpoint for analysis for patients in our cohort. Censored data (all censored data in patient subset showed no biochemical recurrence) are for the last documented follow-up. Log-rank test was performed to assess statistical significance between survival curves. A P -value <0.05 was considered statistically significant. Kaplan–Meier survival analysis was also carried out for two independent patient cohorts, TMA2 and TMA5 ( Supplementary Data 1 and 2 ). TMA2 and TMA5 were obtained from New York University and University of Chicago, respectively, through Cooperative Prostate Cancer Tissue Resource. TMA5 is a large patient cohort that was organized according to the biochemical recurrence of PC. Biochemical recurrence in Cooperative Prostate Cancer Tissue Resource was defined as an increase in serum PSA levels >0.6 ng ml −1 (single value) or consecutive rise in serum PSA levels between 0.4 and 0.6 ng ml −1 after radical prostatectomy [57] . Tissue microarray staining and analysis TMA2 was organized according to Gleason score and consisted of 1,128 PC tissue cores that were derived from 250 patients ( Supplementary Data 1 ). TMA5 contained 1,616 PC tissue cores that were derived from 404 patients based on their PC biochemical recurrence ( Supplementary Data 2 ). IHC staining of TMA was performed according the procedure described above. TMA slides were scanned using a ScanScope (University of Toronto) and analysed using the ImageScope software. All spots (stained cores) were also manually examined to exclude those spots that were either scratched or contained no prostate glands (only stromal tissue). All spots were also manually scored. The scores obtained using the ImageScope software are identical with the scores obtained manually. Statistical analysis was performed as described below. Statistical analysis Statistical analysis was performed using SPSS 10.0 for Windows software. For immunohistochemical analysis, Pearson's ϕ coefficient (Pearson's r computed on two dichotomous variables) was used to test for correlations between MAN2C1 and PTEN, and between MAN2C1 and AKT pSer473 (AKT-P) in normal, PIN and carcinoma. For Kaplan–Meier survival analysis, log-rank test was performed to assess statistical significance between survival curves. All tests were two tailed. For multiple comparisons between normal, PINs and different PC Gleason scores, a one-way ANOVA was performed. A P -value <0.05 was considered statistically significant for all tests. How to cite this article: He, L. et al . α-Mannosidase 2C1 attenuates PTEN function in prostate cancer cells. Nat. Commun. 2:307 doi: 10.1038/1309 (2011).